Theindicanitrate reductase geneOsNR2allele enhances rice yield potential and nitrogen use efficiency The indica and japonica rice ( Oryza sativa ) subspecies differ in nitrate (NO 3 − ) assimilation capacity and nitrogen (N) use efficiency (NUE). Here, we show that a major component of this difference is conferred by allelic variation at OsNR2 , a gene encoding a NADH/NADPH-dependent NO 3 − reductase (NR). Selection-driven allelic divergence has resulted in variant indica and japonica OsNR2 alleles encoding structurally distinct OsNR2 proteins, with indica OsNR2 exhibiting greater NR activity. Indica OsNR2 also promotes NO 3 − uptake via feed-forward interaction with OsNRT1.1B , a gene encoding a NO 3 − uptake transporter. These properties enable indica OsNR2 to confer increased effective tiller number, grain yield and NUE on japonica rice, effects enhanced by interaction with an additionally introgressed indica OsNRT1.1B allele. In consequence, indica OsNR2 provides an important breeding resource for the sustainable increases in japonica rice yields necessary for future global food security. Two distinct cultivated indica and japonica subspecies arose during Asian rice domestication [1] , [2] . Indica - and japonica -type cultivars can be reliably distinguished using characteristic traits [3] , [4] , [5] , among which is relative resistance to toxic chlorate (ClO 3 − ) ion. However, while the genes underlying several of these distinguishing traits have been mapped or molecularly cloned [6] , [7] , [8] , [9] , [10] , [11] , the molecular and evolutionary causes of differential rice ClO 3 − resistance [12] remain unclear. ClO 3 − is relatively toxic to rice and other plants because it is a NO 3 − analog [13] . Soil NO 3 − is absorbed through specific root uptake transporters [14] , and subsequently reduced to nitrite (NO 2 − ) by the NR enzyme of NO 3 - assimilation [15] . The ClO 3 − is absorbed by NO 3 − uptake transporters, and then reduced by NR to the toxic chlorite (ClO 2 − ), which inhibits plant growth. Accordingly, mutants deficient in NO 3 − uptake transporter or NR function are relatively ClO 3 − resistant [16] , [17] . Rice is mostly cultivated in anaerobic paddy field soils, where ammonium (NH 4 + ) rather than NO 3 − predominates as N source. Nevertheless, specialized aerenchyma rice root cells transfer oxygen from shoot to root, causing release into the rhizosphere. The resultant enhancement of soil bacterial conversion of NH 4 + to NO 3 − (nitrification) [18] provides 15–40% of paddy field grown rice N uptake [19] . The efficiency of NO 3 − uptake and assimilation is therefore a key effector for paddy-grown rice productivity, and variation in ClO 3 − resistance is a valuable proxy indicator for relative rice NO 3 − assimilation efficiencies. Here, we identify major quantitative trait loci (QTLs) conferring the ClO 3 − resistance differences between the indica (variety 9311) and japonica (Nipponbare) rice subspecies. Fine mapping, molecular cloning, and further analyses show one of these QTLs ( qCR2 ) to encode the NAD(P)H-dependent nitrate reductase (NR) OsNR2. We also show that a key arginine residue (Arg 783 ) in the NAD(P) binding domain of the 9311 ( indica ) OsNR2 confers a specific NR activity greater than that of the Nipponare ( japonica ) OsNR2, in which a Trp residue is substituted for Arg 783 . Further phylogenetic and evolutionary analyses suggest that allelic divergence at OsNR2 has been driven by directional selection on both indica and japonica alleles. Finally, we show that the indica OsNR2 allele confers superior grain yield and NUE (versus the japonica allele), in part via feed-forward interaction with OsNRT1.1B , a gene coding for a NO 3 − uptake transporter [20] . OsNR2 is a major determinant of rice ClO 3 − resistance Six major ClO 3 − resistance QTLs were detected in analysis of recombinant inbred line (RIL) seedlings from a 9311 ( indica ) × Nipponbare (NPB, japonica ) cross (Fig. 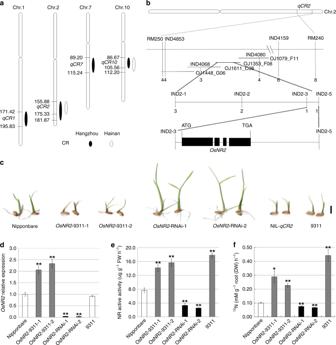Fig. 1 OsNR2allelic variation confers theqCR2, and affects NR active activity and15NO3- uptake.aClO3−resistance (CR) QTL analysis of RILs from anindica(9311) ×japonica(Nipponbare) cross, performed on seedlings germinated from seeds harvested in Hangzhou or Hainan (see Methods). Major QTLs are shown, with numbers indicating genetic map position (cM) on each chromosome.bFine mapping ofqCR2with a residual heterozygote line (RHL) F2population. Using a panel of linked markers (Supplementary Table2),qCR2was pin-pointed to a 6.4 kb region (Chr.2, between markers IND2-3 and IND2-5) containingOsNR2. Numbers of recombinants between each marker andqCR2are shown.OsNR2structure is shown, black boxes represent exons.cRelative seedling vigor indicates degree of ClO3−resistance (Nipponbare harboring constructs for expression of the 9311OsNR2allele driven by the 9311OsNR2promoter (OsNR2-9311-1 andOsNR2-9311-2) or ofOsNR2RNAi (OsNR2-RNAi-1 andOsNR2-RNAi-2); see Supplementary Fig.1).dLeafOsNR2mRNA abundance,eleaf NR active activity,f15NO3−uptake activity of roots exposed to 1.25 mM15NO3−. Value is mean ± s.d. (n= 3 ford–f). Error bar represents s.d. * and ** respectively indicate least significant differences at the 0.05 and 0.01 probability level compared with Nipponbare. The source data underlying Fig.1d–fare provided as a Source Data file 1a and Supplementary Table 1 ). Of these, the map positions of qCR2 and qCR10 correspond with previously identified ClO 3 − resistance QTLs [21] , with qCR10 reflecting variation at OsNRT1.1B , a gene encoding a NO 3 - uptake transporter [20] . Because qCR2 is a strong ClO 3 − resistance QTL (with PVE of 8.0 in Hangzhou (HZ) and 23.8 in Hainan (HN), Supplementary Table 1 ), we delimited it to a single candidate OsNR2 gene (see Methods, Fig. 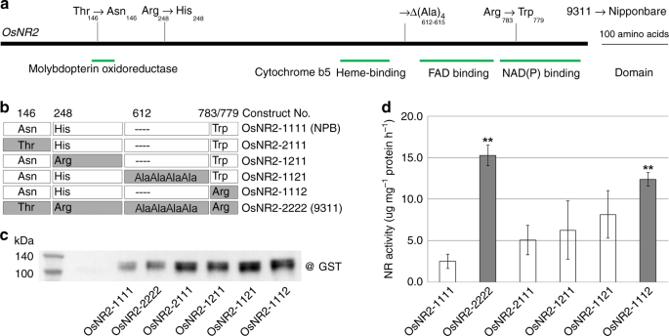Fig. 2 An Arg-Trp amino acid substitution reduces the specific activity of Nipponbare OsNR2.aAmino acid substitution and insertion differences between the 9311 and Nipponbare OsNR2 proteins. Locations of conserved functional domains are indicated by green bars.bConstructs expressing chimeric OsNR2 proteins of varying amino acid sequence. Fragments from the 9311 and Nipponbare OsNR2 coding regions were exchanged to generate constructs encoding a series of four different chimeric OsNR2 proteins, differing with respect to the amino acid residues variant between 9311 and Nipponbare OsNR2. These constructs were expressed inE.coli.cDetection with anti:GST antibody (Cat No: CW0084M, CWBIOtech, Beijing, China) of OsNR2-GST fusion proteins extracted fromE. coliand purified on a GST-sefinoseTMcolumn (constructs as shown inb), showing roughly equivalent abundance of OsNR2 proteins.dNR activity of purified extracts as inb,c. Value is mean ± s.d. (n= 3). Error bar represents s.d. ** indicates the least significant difference at 0.01 probability level compared with Nipponbare. The source data underlyingcanddare provided as a Source Data file 1b and Supplementary Table 2 ). OsNR2 encodes OsNR2, a NAD(P)H-dependent nitrate reductase (NR) ( http://rice.plantbiology.msu.edu/ ) having dual ability to accept both NADPH and NADH as electron donors [22] . Expression of the 9311 OsNR2 allele (driven by the 9311 OsNR2 promoter) in Nipponbare increases ClO 3 − sensitivity (Fig. 1c and Supplementary Fig. 1a ), while reduction of OsNR2 mRNA abundance increases Nipponbare ClO 3 − resistance (Figs. 1 c, 1d ; Supplementary Fig. 1b ), thus confirming that allelic variation at OsNR2 is causal of qCR2 . Fig. 1 OsNR2 allelic variation confers the qCR2 , and affects NR active activity and 15 NO 3 - uptake. a ClO 3 − resistance (CR) QTL analysis of RILs from an indica (9311) × japonica (Nipponbare) cross, performed on seedlings germinated from seeds harvested in Hangzhou or Hainan (see Methods). Major QTLs are shown, with numbers indicating genetic map position (cM) on each chromosome. b Fine mapping of qCR2 with a residual heterozygote line (RHL) F 2 population. Using a panel of linked markers (Supplementary Table 2 ), qCR2 was pin-pointed to a 6.4 kb region (Chr.2, between markers IND2-3 and IND2-5) containing OsNR2 . Numbers of recombinants between each marker and qCR2 are shown. OsNR2 structure is shown, black boxes represent exons. c Relative seedling vigor indicates degree of ClO 3 − resistance (Nipponbare harboring constructs for expression of the 9311 OsNR2 allele driven by the 9311 OsNR2 promoter ( OsNR2 -9311-1 and OsNR2 -9311-2) or of OsNR2 RNAi ( OsNR2- RNAi-1 and OsNR2- RNAi-2); see Supplementary Fig. 1 ). d Leaf OsNR2 mRNA abundance, e leaf NR active activity, f 15 NO 3 − uptake activity of roots exposed to 1.25 mM 15 NO 3 − . Value is mean ± s.d. ( n = 3 for d – f ). Error bar represents s.d. * and ** respectively indicate least significant differences at the 0.05 and 0.01 probability level compared with Nipponbare. The source data underlying Fig. 1d–f are provided as a Source Data file Full size image A dose experiment for nitrate reductase activity in different concentration of nitrate and NADPH showed NR active activity of Nipponbare and 9311 were dependent on KNO 3 concentration and NADPH concentration, respectively (Supplementary Fig. 2a , 2b ). Therefore, 5 mM KNO 3 and 0.2 mM NADPH were selected for NR activity assay. 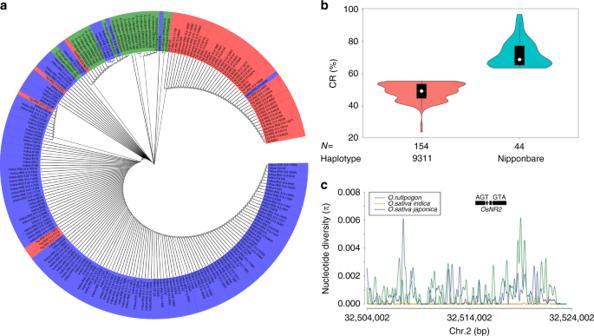Fig. 3 Phylogenetic and functional analysis ofOsNR2haplotypes.aPhylogenetic tree ofOsNR2CDS from 222 accessions. Blue:O. sativa indica; red:O. sativa japonica; green:O. rufipogon; Tej:Temperate japonica; Trj:Tropical japonica.bClassification of 199 cultivated rice varieties according to haplotype (9311 versus Nipponbare) and extent of conferred ClO3-resistance (CR%). Error bars represent 95% confidence intervals.cDNA sequence diversity of the genomic region surroundingOsNR2in three groups. The green, orange and blue lines indicate site nucleotide diversity (π) forO. rufipogon,O. sativa indicaandO. sativa japonicaaccessions, respectively. The position ofOsNR2is as indicated (thick lines represent exons and thin lines introns). The source data underlying b are provided as a Source Data file Km of NR active activity for NADPH and nitrate in Nipponbare were higher than those in 9311 (Supplementary Table 3 ), suggesting allelic variation at OsNR2 may affect binding ability with NADPH and NO 3 − . We also found that expression of 9311 OsNR2 coding sequence or reduction in OsNR2 mRNA abundance respectively caused increase or decrease in Nipponbare maximal and active NR activity (Fig. 1 e, Supplementary Fig. 2c ), changes in enzymatic activity that mirror the effect of allelic variation at OsNR2 on relative ClO 3 − resistance. In addition, expression of 9311 OsNR2 coding sequence or reduction in OsNR2 mRNA abundance caused intriguing parallel effects on NO 3 − uptake capacity (Fig. 1f ), with the 9311 OsNR2 allele conferring relative increase in rate of NO 3 − uptake. The Trp 779 substitution reduces japonica OsNR2 activity Despite the differences in conferred ClO 3 − resistance, OsNR2 mRNA abundance does not detectably differ between 9311 and Nipponbare (Fig. 1d ), suggesting that the 9311 OsNR2 protein is intrinsically more active than Nipponbare OsNR2. Accordingly, we found that 9311 and Nipponbare OsNR2 protein-encoding regions differ by 3 nonsynonymous SNPs (conferring Thr 146 to Asn 146 , Arg 248 to His 248 and Arg 783 to Trp 779 substitutions; 9311 to Nipponbare respectively) and by a 12-bp indel (conferring deletion of Ala 612-615 from Nipponbare OsNR2; Fig. 2a and Supplementary Fig. 3 ). Because Thr 146 , Arg 248 and Arg 783 (as in 9311 OsNR2) are all strictly conserved in OsNR2 orthologues from related grass species (Supplementary Fig. 4 ), we determined the individual effects of these residues on the activity of E.coli -expressed OsNR2 (Fig. 2b ). Using NADH as electron donor, no significant differrence was found between 9311 and Nipponbare OsNR2 protein (Supplementary Fig. 5 ). Thus, NADPH was then used as the reducer. And we found that a Trp 779 to Arg 783 substituted OsNR2 (OsNR2-1112) exhibited significantly increased NR activity (Fig. 2c, d ). Therefore, the Arg 783 to Trp 779 substitution in the NAD(P) binding domain of Nipponbare OsNR2 (Fig. 2a ) reduces specific NR activity, conferring increased ClO 3 - resistance, and indicating that Nipponbare OsNR2 is a reduced function variant allele. Fig. 2 An Arg-Trp amino acid substitution reduces the specific activity of Nipponbare OsNR2. a Amino acid substitution and insertion differences between the 9311 and Nipponbare OsNR2 proteins. Locations of conserved functional domains are indicated by green bars. b Constructs expressing chimeric OsNR2 proteins of varying amino acid sequence. Fragments from the 9311 and Nipponbare OsNR2 coding regions were exchanged to generate constructs encoding a series of four different chimeric OsNR2 proteins, differing with respect to the amino acid residues variant between 9311 and Nipponbare OsNR2. These constructs were expressed in E.coli . c Detection with anti:GST antibody (Cat No: CW0084M, CWBIOtech, Beijing, China) of OsNR2-GST fusion proteins extracted from E. coli and purified on a GST-sefinose TM column (constructs as shown in b ), showing roughly equivalent abundance of OsNR2 proteins. d NR activity of purified extracts as in b , c . Value is mean ± s.d. ( n = 3). Error bar represents s.d. ** indicates the least significant difference at 0.01 probability level compared with Nipponbare. The source data underlying c and d are provided as a Source Data file Full size image OsNR2 allelic divergence was driven by selection Phylogenetic analyses of O.sativa indica , O.sativa japonica and O. rufipogon accessions next determined the extent to which the 9311 and Nipponbare OsNR2 alleles are representative of overall indica versus japonica OsNR2 divergence (Fig. 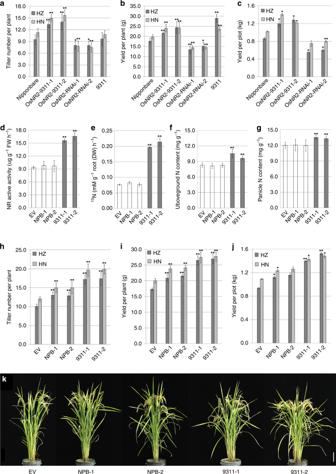Fig. 4 Expression of the 9311OsNR2allele boosts Nipponbare N assimilation, tiller number, and grain yield.aeffective tiller number,byield per plant andcyield per plot of Nipponbare, Nipponbare harboring constructs for expression of the 9311OsNR2allele driven by the 9311OsNR2promoter (OsNR2-9311-1 andOsNR2-9311-2) or ofOsNR2RNAi (OsNR2-RNAi-1 andOsNR2-RNAi-2).dNR active activity of Nipponbare (empty-vector control; EV), transgenic derivatives expressing the 9311OsNR2allele (9311-1 and 9311-2), and transgenic derivatives expressing the NipponbareOsNR2allele (NPB-1 and NPB-2), with expression of both alleles being driven by the CaMV 35S promoter.e15NO3-uptake of plants exposed to 1.25 mM15NO3,fN content of aboveground plant parts,gpanicle N content,heffective tiller number,iyield per plant,jyield per plot andkappearance of plant genotypes (as in (d)). Plants were cultivated in field conditions with NO3−fertilizer (14 kg per acre) as major N sourcef–i. Values are mean ± s.d. (n= 6 fora-b,f–i,n= 3 ford,eandn= 2 forc,j). Error bar represents s.d. * and ** respectively indicate least significant differences at the 0.05 and 0.01 probability levels, compared with Nipponbare or EV. HZ: Hangzhou (harvested on September 20th, 2018); HN: Hainan (harvested on April 20th, 2019). Source data are provided as a Source Data file 3a ) by F st value (Supplementary Table 4 ). Further analysis of cultivated varieties identified two distinct OsNR2 haplotypes defined by the three nonsynonymous SNPs distinguishing the 9311 and Nipponbare OsNR2 alleles (Fig. 2a ; Supplementary Fig. 3 ). Almost all indica varieties (147 of 148) carry the 9311 haplotype (conferring ClO 3 − sensitivity), while most japonica varieties (43 of 51, including both temperate and tropical varieties) carry the Nipponbare haplotype (conferring ClO 3 − resistance) (Fig. 3b ). Thus, the 9311 versus Nipponbare OsNR2 alleleic difference is largely reflective of overall indica versus japonica OsNR2 allelic divergence, explaining why indica and japonica cultivars can be reliably distinguished in ClO 3 − resistance assays. Fig. 3 Phylogenetic and functional analysis of OsNR2 haplotypes. a Phylogenetic tree of OsNR2 CDS from 222 accessions. Blue: O. sativa indica ; red: O. sativa japonica ; green: O. rufipogon ; Tej: Temperate japonica ; Trj: Tropical japonica . b Classification of 199 cultivated rice varieties according to haplotype (9311 versus Nipponbare) and extent of conferred ClO 3 - resistance (CR%). Error bars represent 95% confidence intervals. c DNA sequence diversity of the genomic region surrounding OsNR2 in three groups. The green, orange and blue lines indicate site nucleotide diversity (π) for O. rufipogon , O. sativa indica and O. sativa japonica accessions, respectively. The position of OsNR2 is as indicated (thick lines represent exons and thin lines introns). The source data underlying b are provided as a Source Data file Full size image Nucleotide diversity (π) analysis of OsNR2 and neighboring regions (10 kb) showed reduction of 99.0% ( indica ) or 96.0% ( japonica ) of O. rufipogon OsNR2 diversity, indicating that directional selection [23] , [24] has driven the evolutionary divergence of the indica and japonica OsNR2 alleles (Fig. 3c ). Correspondingly, a neutrality test [25] detected significant selection signatures for both alleles (Tajima’s D -1.96 for indica versus −2.11 for japonica ; P < 0.05), the evidence of selective sweeps. Total of 100 genes were randomly selected from the sequenced japonica and indica genomes and average nucleotide diversity was calculated. The OsNR2 nucleotide diversity was 9.06-fold and 3.75-fold lower than that of 100 randomly chosen gene fragments in the indica (π = 0.00280) and japonica (π = 0.00282) sample, respectively (Supplementary Data 1 ), suggesting that the lower nucleotide diversity observed in OsNR2 loci of indica and japonica resulted from strong selection of it occurred during rice domestication. Furthermore, most japonica varieties (42 of 50) exhibited a ka/ks > 1, indicating that positive selection drove the divergence of the japonica OsNR2 allele (Supplementary Fig. 6 ), despite its relatively reduced conferred NR function. The 9311 OsNR2 allele promotes grain yield pOsNR2-GUS fusion construct and qRT-PCR experiments indicated OsNR2 was expressed in shoot and root vasculature, young root elongation zones, flowers and mostly in leaf (Supplementary Fig. 7 ). We next determined the effects of expression of the 9311 OsNR2 allele on agronomic traits. First, we found that effective tiller number is respectively increased or decreased in Nipponbare plants expressing 9311 OsNR2 (expression driven by the 9311 OsNR2 promoter) or having reduced OsNR2 mRNA abundance in Hangzhou (HZ) and Hainan (HN) (Fig. 4a , Supplementary Fig. 8 ). Correspondingly, the transcript abundances of OsTB1 [26] , a gene controlling tiller bud formation and elongation, was reduced by expression of 9311 OsNR2 , but increased by reduction in OsNR2 mRNA abundance (Supplementary Fig. 9 ). Second, with effective tiller number being an important contributor to yield, we found that yield per plant and yield per plot in both HZ and HN were respectively increased or decreased in Nipponbare plants expressing 9311 OsNR2 or having reduced OsNR2 mRNA abundance (Fig. 4b, c ). We next found that transgenic expression of the 9311 OsNR2 allele (driven by the CaMV 35S promoter) increased the maximal and active NR activity, 15 NO 3 − uptake activity, and aboveground and panicle nitrogen contents of Nipponbare plants (9311-1 and 9311-2; Fig. 4d–g ; Supplementary Fig. 2d ). Transgenic expression of the 9311 OsNR2 allele also conferred increased effective tiller number and grain yield on Nipponbare grown with NO 3 − as the major N source in both HZ and HN, while Nipponbare effective tiller number and yield were also increased by transgenic expression of the Nipponbare OsNR2 allele, these effects were not as great as seen with the 9311 allele (Fig. 4 h–k, Supplementary Fig. 10a ). Fig. 4 Expression of the 9311 OsNR2 allele boosts Nipponbare N assimilation, tiller number, and grain yield. a effective tiller number, b yield per plant and c yield per plot of Nipponbare, Nipponbare harboring constructs for expression of the 9311 OsNR2 allele driven by the 9311 OsNR2 promoter ( OsNR2 -9311-1 and OsNR2 -9311-2) or of OsNR2 RNAi ( OsNR2- RNAi-1 and OsNR2- RNAi-2). d NR active activity of Nipponbare (empty-vector control; EV), transgenic derivatives expressing the 9311 OsNR2 allele (9311-1 and 9311-2), and transgenic derivatives expressing the Nipponbare OsNR2 allele (NPB-1 and NPB-2), with expression of both alleles being driven by the CaMV 35S promoter. e 15 NO 3 - uptake of plants exposed to 1.25 mM 15 NO 3 , f N content of aboveground plant parts, g panicle N content, h effective tiller number, i yield per plant, j yield per plot and k appearance of plant genotypes (as in ( d )). Plants were cultivated in field conditions with NO 3 − fertilizer (14 kg per acre) as major N source f – i . Values are mean ± s.d. ( n = 6 for a - b , f – i , n = 3 for d , e and n = 2 for c , j ). Error bar represents s.d. * and ** respectively indicate least significant differences at the 0.05 and 0.01 probability levels, compared with Nipponbare or EV. HZ: Hangzhou (harvested on September 20th, 2018); HN: Hainan (harvested on April 20th, 2019). Source data are provided as a Source Data file Full size image Feed-forward interaction of OsNR2 with OsNRT1.1B Because qCR2 ( OsNR2 ) and qCR10 ( OsNRT1.1B [20] ) have strong individual effects on ClO 3 − resistance, we next investigated their inter-relationships and found that the 9311 OsNR2 allele increases OsNRT1.1B mRNA abundance in both NIL- qCR2 (Fig. 5a ) and transgenics (Supplementary Fig. 10b ). These observations suggest that the increased NO 3 − uptake conferred by 9311 OsNR2 (Figs. 1f and 4e ) may be due to increased OsNRT1.1B activity. Reciprocally, the indica OsNRT1.1B allele (in NIL- qCR10 ) confers increased OsNR2 mRNA abundance and enhanced NR activity (Fig. 5b, c ). These observations imply a feed-forward amplifying relationship, with OsNR2 function promoting OsNRT1.1B function, and vice versa . Indeed, a double Nipponbare NIL carrying both of the indica OsNRT1.1B and OsNR2 alleles (NIL- qCR2/qCR10 ) displayed increased OsNRT1.1B and OsNR2 mRNA abundances and NR activity above those of either single NIL (NIL- qCR2 or NIL- qCR10 ) (Fig. 5a-c ), resulting in NIL- qCR2/qCR10 having the highest NO 3 − uptake, aboveground N content, panicle N content, effective tiller number and yield per plant in both HZ and HN (Supplementary Fig. 11 ; Fig. 5e-f ). The yield-enhancing increased effective tiller number of NIL- qCR2/qCR10 is associated with corresponding decreases in OsTB1 (Supplementary Fig. 12 ). Further analysis showed that the root 15 NO 3 − uptake activity and OsNRT1.1B mRNA abundance of all tested indica varieties is significantly higher than that of japonica varieties (Supplementary Fig. 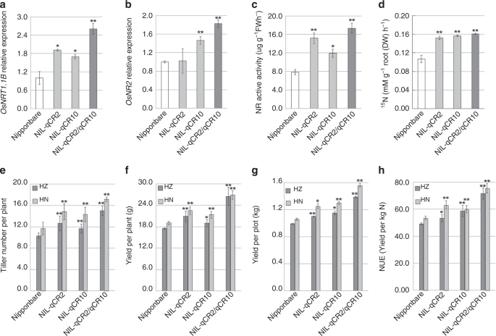Fig. 5 OsNR2andOsNRT1.1Binteract to promote rice yield and NUE.arootOsNRT1.1BmRNA abundance,bleafOsNR2mRNA abundance,cleaf NR active activity,d15NO3−uptake activity of roots exposed to 1.25 mM15NO3−,eeffective tiller number,fyield per plant,gyield per plot andhNUE of Nipponbare, NIL-qCR2, NIL-qCR10and NIL-qCR2/qCR10. Values are mean ± s.d. (n= 3 fora–d,n= 6 fore,f,handn= 2 forg). Error bar represents s.d. Plants cultivated in field conditions with NO3−fertilizer (14 kg per acre) as major N sourcee–h. * and ** respectively indicate least significant differences at the 0.05 and 0.01 probability levels, compared with Nipponbare. HZ: Hangzhou (harvested on September 20th, 2018); HN: Hainan (harvested on April 20th, 2019). Source data are provided as a Source Data file 13 ; Supplementary Table 5 ), further strengthening the conclusion that there is a feed-forward relationship between OsNR2 and OsNRT1.1B . Finally, urea-fertilized (180 kg N ha −1 ) paddy field experiments again revealed NIL- qCR2/qCR10 to have the highest yield per plot and NUE in HZ (cultivated from May to September, 2018) and HN (cultivated from December, 2018 to April, 2019) versus Nipponbare, NIL- qCR2 or NIL- qCR10 (Fig. 5g, h ). Fig. 5 OsNR2 and OsNRT1.1B interact to promote rice yield and NUE. a root OsNRT1.1B mRNA abundance, b leaf OsNR2 mRNA abundance, c leaf NR active activity, d 15 NO 3 − uptake activity of roots exposed to 1.25 mM 15 NO 3 − , e effective tiller number, f yield per plant, g yield per plot and h NUE of Nipponbare, NIL- qCR2 , NIL- qCR10 and NIL- qCR2/qCR10 . Values are mean ± s.d. ( n = 3 for a – d , n = 6 for e , f , h and n = 2 for g ). Error bar represents s.d. Plants cultivated in field conditions with NO 3 − fertilizer (14 kg per acre) as major N source e – h . * and ** respectively indicate least significant differences at the 0.05 and 0.01 probability levels, compared with Nipponbare. HZ: Hangzhou (harvested on September 20th, 2018); HN: Hainan (harvested on April 20th, 2019). Source data are provided as a Source Data file Full size image We have shown that allelic variation at OsNR2 underlies the ClO 3 − resistance QTL qCR2 , and that OsNR2 encodes a NAD(P)H-bispecific NR enzyme. Whilst NADH-specific NRs are relatively well understood [27] , little is known about the function of NAD(P)H-bispecific NRs in rice. Nevertheless, we have here shown that the OsNR2 (here NADPH mainly specific) is actually a major contributor to rice ClO 3 − resistance, grain yield and NUE. Specifically, we have shown that the Arg 783 residue characteristic of the NAD(P) binding domain of 9311 OsNR2 (but replaced by Trp 779 in Nipponbare OsNR2) is responsible for the greater ClO 3 - sensitivity and active NR activity conferred by 9311 OsNR2 (versus that conferred by Nipponbare OsNR2 ) (Fig. 2 ). In our study, haplotype analysis indicated that the 9311 and Nipponbare OsNR2 alleles are largely representative of overall differences between indica and japonica OsNR2 alleles. Phylogenetic analysis also indicated grouping of indica OsNR2s together with those from O.rufipogon accessions, suggesting greater divergence of japonica OsNR2 from the presumed ancestral wild rice OsNR2 (Fig. 3a ). Furthermore, our ka/ks ratio analysis revealed evidence of positive selection [28] , with OsNR2 exhibiting a ka/ks > 1 in 42 out of 50 japonica varieties (Supplementary Fig. 6 ). Thus, despite being a reduced function allele, japonica OsNR2 was under positive selection during the differentiation of indica and japonica , perhaps during adaptation to distinct climatic, ecogeographic or cultural conditions. However, the correspondence between haplotype and varietal identity is not absolute, with several japonica varieties carrying the 9311 OsNR2 haplotype and a single indica variety carrying the Nipponbare OsNR2 haplotype. Nevertheless, ClO 3 − resistance correlates strictly with OsNR2 haplotype (Fig. 3b ), further highlighting the key role of the Arg 783 residue of 9311 OsNR2. We have also identified a previously unknown regulatory relationship between OsNR2 nitrate reductase and OsNRT1.1B NO 3 – uptake transporter functions in rice, showing that the 9311 OsNR2 allele increases OsNRT1.1B function, while the 9311 OsNRT1.1B allele also increases OsNR2 function. While reciprocal regulation of NO 3 − uptake and assimilation functions have previously been described in Arabidopsis [29] , [30] , [31] , there are potentially differences between Arabidopsis and rice in the specifics of their relationships. Further work will define in greater depth the nature of the feed-forward interaction between OsNR2 and OsNRT1.1B . Effective tiller number is an important contributory component of rice grain yield, and correlates positively with soil N availability [32] , with leaf and sheath N content influencing tiller emergence [33] . Although yield per plant of 9311 is significantly higher than Nipponbare both in HZ and HN, tiller number are similar between them (Fig. 4a, b ). Therefore, increase in effective tiller number conferred by 9311 OsNR2 allele was dependent on genetic background. Here, we have shown that the greater N-assimilative NR activity of indica OsNR2 (versus japonica OsNR2) confers enhanced tiller number, grain yield and NUE (Fig. 5c, e–h ). In conclusion, indica OsNR2 has greater specific activity than the diverged japonica OsNR2, and hence boosts the chlorate sensitivity 15 NO 3 − uptake and grain yield of indica varieties. NUE is further enhanced by the promotive feed-forward amplifying functional relationship between the indica OsNRT1.1B and OsNR2 alleles, and this is particularly evident following introgression of both alleles into japonica varieties. Genetic variation at both OsNR2 and OsNRT1.1B should therefore become major targets for breeders aiming to improve the world’s rice yield and the prospects for future global food security. Development of plant materials and molecular markers A total of 152 recombinant inbred lines (RILs) were derived from crossing the japonica variety Nipponbare with the indica variety 9311. These populations were subsequently developed in experimental fields at the China National Rice Research Institute in Hangzhou, Zhejiang Province, and in Lingshui, Hainan Province, China. To develop the NIL for the qCR2 QTL (detected both in Hainan and Hangzhou), a RIL carrying the 9311 genotype in the qCR2 region was selected for recurrent backcrossing with Nipponbare. SSR markers RM240 and RM250 (Supplementary Table 2 ) were used for marker-assisted selection (MAS) in each generation. As a result, a BC 4 F 1 line, with a substantially Nipponbare genetic background but heterozyogous for DNA from 9311 and Nipponbare across the qCR2 region was identified. Following self-pollination, derived BC 4 F 2 and BC 4 F 3 populations were obtained and used for the fine mapping of qCR2 . Additionally, two NILs homozygous for 9311 DNA in the target QTL region between InDel markers IND2-1 and IND2-5, and SSR markers RM3123 and RM5666 (Supplementary Table 2 ) were respectively developed in the Nipponbare background and designated NIL- qCR2 and NIL- qCR10 . Subsequently, NIL- qCR2/qCR10 was screened from the F 2 of a cross between NIL- qCR2 and NIL- qCR10 . For the haplotype and phylogenetic analyses, 199 cultivated rice accessions were sampled, including 148 O. sativa indica and 51 O. sativa japonica accessions. All varieties were from the China National Rice Research Institute (Hangzhou, China) or the International Rice Research Institute (Philippines). Additional 23 O.rufipogon rice accessions were also sampled (Supplementary Table 6 ). Determination of ClO 3 - resistance ClO 3 − resistance phenotypes were investigated at the seedling germination stage, using a method based on that described in Teng et al. [21] . Briefly, rice seeds were placed in a petri-dish on filter paper fully wetted with distilled water or with a 0.02% potassium chlorate solution, and then incubated at 28 °C, 14h-light/10h-dark period (RXZ-500D, Ningbo Jiangnan Instrument, China). The solution was changed every other day. In total 12 seedlings were measured in each sample, with ClO 3 − resistance phenotypes being determined after 7 days (by measuring the length of each seedling). ClO 3 − resistance was calculated as the following Equation 1 : ClO 3 − resistance (CR %) = (Average seedling length in ClO 3 − /Average seedling length in water) × 100%. ( 1 ). QTL mapping A genetic map consisting of 134 InDel and SSR markers evenly distributed throughout the 12 rice chromosomes was constructed for QTL mapping. QTL analysis was performed with the MultiQTL package (www.multiqtl.com), using the maximum likelihood interval mapping approach for the RIL-selfing population. For major-effect QTLs, the LOD threshold was obtained based on a permutation test (1000 permutations) for each dataset. QTLs were named according to McCouch et al. [34] . DNA extraction and OsNR2 sequencing Genomic DNA was extracted from fresh rice leaves using the cetyl-trimethyl-ammonium bromide (CTAB) method [35] , with minor modifications. To obtain the OsNR2 genomic DNA sequence, a 3026-bp region of the OsNR2 gene from the start ATG to the TGA was amplified with LA Taq DNA polymerase in GC buffer I (Takara), using PCR sequencing primers NR3-NR8 (Supplementary Table 7 ). The PCR products were purified with a purification kit (Tiangen Company). All PCR products were sequenced directly on both strands with the primers. SNP calling, phylogenetic and genetic diversity analysis We downloaded genome sequence data of 222 rice accessions from previous studies [36] , [37] , [38] . Rice reference genome (MSU v7.0) was downloaded from the Rice Genome Annotation Project ( http://rice.plantbiology.msu.edu/pub/data/Eukaryotic_Projects/o_sativa/annotation_dbs/pseudomolecules/version_7.0/all.dir/ ). The genome sequence data of 147 O.sativa indica and 50 O. sativa japonica were obtained from NCBI ( https://www.ncbi.nlm.nih.gov/biosample?Db=biosample&DbFrom=bioproject&Cmd=Link&LinkName=bioproject_biosample&LinkReadableName=BioSample&ordinalpos=1&IdsFromResult=262761 ). The sequence data of 23 O. rufipogon were downloaded from the NCBI BioProject PRJEB19404 ( https://www.ncbi.nlm.nih.gov/bioproject/?term=PRJEB19404 ; ERR2240123, ERR2240125, ERR2240126, ERR2245548-ERR2245557), PRJDA39855 ( https://www.ncbi.nlm.nih.gov/bioproject/?term=PRJDA39855 ; DRR000347, DRR000348) and PRJDB2009 ( https://www.ncbi.nlm.nih.gov/bioproject/?term=PRJDB2009 ; DRR001183-DRR001190). Raw reads were trimmed with trimmomatic version 0.36 ( http://www.usadellab.org/cms/uploads/supplementary/Trimmomatic/Trimmomatic-Src-0.36.zip ) with parameters (ILLUMINACLIP:2:30:10 MINLEN:50 LEADING:20 TRAILING:20 SLIDINGWINDOW:5:20), and then aligned to the Nipponbare v7 reference genome ( http://rice.plantbiology.msu.edu/ ) using BWA-MEM v0.7.10 [39] . SNP calling and filtration were carried out with SAMtools version 1.6 (DP < 3 and a quality score < 30) [40] . SNP data from the OsNR2 genomic sequences of 199 cultivated rice and 23 wild rice accessions are supplied in Supplementary Data 2 - 4 . The SNP information from LOC_Os02g53130 CDS was used to generate a maximum likehood phylogeny using MEGA version 5.0 [41] with bootstrap method and 1000 replications. Online tool EvolView version 2 ( http://www.evolgenius.info/evolview/ ) [42] was used to display the phylogenetic tree and for annotation. Calculation of population differentiation extent was estimated by R/Hierfstat package v0.04-22 using the F st statistic [43] , with a 100-kb sliding window with 10-kb steps. Sequence diversity (π) and Tajima’s D were computed with DnaSP v6 [44] for each O. sativa japonica , O. sativa indica and O. rufipogon group [45] . Sequences were aligned by MAFFT (default parameters) and ka/ks value was computed using the Ka/Ks calculator 2.0 [28] . Nucleotide diversity (π) of OsNR2 and 100 randomly selected gene fragments were calculated with vcftools v0.1.13 ( https://sourceforge.net/projects/vcftools/files/ ) [46] with parameter (–site-pi) for indica and japonica groups. Sequence alignments were performed using ClustalX 2.0 [47] . A PCR marker CR2-ID for InDel 2194 is listed in Supplementary Table 7 . Vector construction and plant transformation A 9.773-kb 9311 genomic DNA fragment containing the entire OsNR2 gene, 5356 bp of upstream sequence, and 1378 bp of downstream sequence was amplified with a high-fidelity DNA polymerase. This fragment was inserted into binary vector pCAMBIA1300, thus generating the transformation plasmid pCAMBIA1300- OsNR2 -9311 that was used for the complementation test (Supplementary Fig. 1a ). For plant transformation, the binary plasmid was first introduced into Agrobacterium tumefaciens EHA105 by electroporation, followed by transformation of Nipponbare callus [48] . Hyg primers for hygromycin resistance were used in the screening of transgenic plants (Supplementary Table 7 ). For RNAi analysis, Nipponbare was transformed with pTCK303- OsNR2 -RNAi (Supplementary Fig. 1b ), which contains nucleotides 1–119 of the OsNR2 CDS amplified using the NR2RNAi primer (Supplementary Table 7 ). In addition, a 1.541-kb promoter fragment from Nipponbare OsNR2 was amplified by high fidelity DNA polymerase using NR2P primers (Supplementary Table 7 ) and then inserted upstream of the 5 end of the uidA gene (encoding β-glucuronidase (GUS)) in pCAMBIA1301 (Supplementary Fig. 5a ). The resultant pCAMBIA1301- OsNR2p :GUS fusion vector was transformed into Nipponbare via Agrobacterium tumefaciens . Expression and purification of OsNR2-GST fusion protein The 5 ml overnight cultures of E.coli harboring GST-fusion protein expression constructs were added to 500 ml 2XTY medium with 150 mg ml −1 of ampicillin. The cultures were then shaken at 37 °C until reaching an A 600 of 0.6, at which point protein expression was induced with 0.1 mM of IPTG. The cells were then pelleted 2 h after induction by centrifugation at 2655 × g , 4 °C for 10 min. The supernatant was discarded and the cells re-suspended in 10 ml ice-cold PBS. Next, 200 μl of freshly prepared 10 mg ml -1 lyozyme solution, 4 μl 20 μg ml −1 DNase I, 100 μl 100 mM L −1 MgCl 2 and 100 μl 0.1 mol L –1 PMSF were added, and the mixture was incubated on ice for 30 min. The mixture was then sonicated with 300 W, at 3 s intervals for 20 min, then centrifuged at 15,294 × g at 4 °C for 10 min to pellet the debris. Next, the supernatant was transferred to a GST-Sefinose TM pre-packed gravity column (Cat No: C600911, Sangon Biotech, Shanghai, China) [49] . In total 5 ml binding/wash buffer was twice added, followed by 2 ml elution buffer, which released the GST-fusion protein, which was then used for western blot analysis and determination of enzyme activity. Western blot analysis and NR activity measurement Proteins were separated by 10% SDS–PAGE and western blotting was performed with Anti GST-Tag Mouse Monoclonal Antibody (1000 × dilution, Cat No: CW0084M, CWBIOtech, Beijing, China) [50] . Calibration curves were constructed using BSA (0.5 mg ml −1 ) as standard in the range from 0 to 20 μl measuring absorbance at 595 nm. The purified NR protein was analyzed by applying standard Bradford assays at 595 nm. Nitrate Reductase (NR) activity was measured as described [51] . Briefly, the reaction mixture contained 0.4 mL GST-fusion protein, 1.2 ml 0.1 mmol L −1 potassium phosphate buffer (pH 7.5), 0.1 mmol L −1 KNO 3 , and 0.4 ml 0.25 mmol L −1 nicotinamide adenine dinucleotide phosphate (NADPH). Controls substituted 0.1 mmol L −1 potassium phosphate buffer (pH 7.5) for the NADPH. After 30 min incubation the NO 2 − produced was colorimetrically measured at 540 nm following addition of 10 g kg −1 sulfanilamide in 2 mol L −1 HCl and 0.2 g kg −1 N-(1-naphthyl)-ethylene-diammonium dichloride (NED). NR activity was expressed as μg NO 2 − mg −1 protein h −1 . Measurement of leaf NR activity For enzyme extraction, leaf samples were harvested between 1400 and 1430 hours and ground in liquid nitrogen, following which 5 ml extraction buffer was added (per 1 g fresh tissue). The extraction buffer contained 25 mmol L −1 potassium phosphate buffer (pH 8.8), 10 mmol L −1 cysteine, and 1 mmol L −1 EDTA. Following continuous grinding until thawing, the supernatant was centrifuged at 20,000 × g for 20 min at 4 °C. NR activity was measured as described in the above paragraph except that the 0.4 ml GST-fusion protein was replaced by 0.4 ml extraction aliquots. NR activity was expressed as μg NO 2 − g −1 FW h −1 . Gene expression analysis A real-time polymerase chain reaction (qPCR) approach was used to measure gene expression levels. Total rice leaf RNA was isolated using a Trizol reagent (Invitrogen Inc.). In total 2 µg DNAase-treated total RNA was reverse-transcribed using Moloney murine leukemia virus (M-MLV) reverse transcriptase (Promega Madison, WI) and Oligo(dT) 18 primers (Promega, Madison, WI). Reverse-transcribed products were diluted to one-twentieth, following which 1 µl of the cDNA template was amplified using qPCR primers. Real time PCR amplification mixtures (10 μl) contained 50 ng template cDNA, 2 × SYBR Green PCR Master Mix (Applied Biosystems), and 200 nM forward and reverse primers. Reactions were performed using an ABI PRISM_7900HT Sequence Detector (Applied Biosystems). The relative expression level for each transcript was obtained by comparison with the expression of the Actin gene. Primers for tested genes and Actin are listed in Supplementary Table 7 . GUS assays Histochemical GUS analysis was performed as described with minor modifications [52] . Briefly, transgenic plant samples were incubated in X-Gluc buffer overnight at 37 °C. The stained tissues were observed and photographed using a stereomicroscope with a camera (Nikon SMZ1000). N content assays For field-based assays, plants were grown at the China National Rice Research Institute with NO 3 − fertilizer (14 kg per acre) as major N source. Fertilizer was applied three times during growth: as basal fertilizer (1–2 days before transplanting), tillering fertilizer (7 days after transplanting) and heading-stage fertilizer. N content was determined with the Auto Kjeldahl Nitrogen Analysis System (UDK152, VELP, Italy) using the Kjeldahl method [53] . 15 NO 3 − uptake activity and 15 N accumulation determination Hydroponic growth conditions for rice seedlings were IRRI culture medium at pH 5.5 but with 1.25 mM KNO 3 as the N supply [54] . Rice seedlings were first grown in this medium for 8 weeks in the greenhouse, and then subsequently deprived of N for 3 days. The plants were then rinsed in 0.1 mM CaSO 4 for 1 min, then transferred to a solution containing 1.25 mM 40% atom 15 NO 3 − (Shanghai Research Institute of Chemical Industry) for 5 min for 15 N influx and 3 days for 15 N accumulation, respectively, finally rinsed again in 0.1 mM CaSO 4 for 1 min. Roots were separated from the shoots immediately following the final transfer to CaSO 4 . Samples were heated at 105 °C for 30 min, and then dried at 75 °C for 3 days. Dry weights were recorded as biomass values. 15 N content measurements were performed by gas isotope mass spectrometer (MAT-271). Uptake activity was calculated as the amount of 15 N taken up per unit weight of roots per unit time. Analyses of agronomic traits Important agronomic traits including effective tiller number per plant and grain yield per plant were measured in Hangzhou and Hainan on a single-plant basis, with 6 plants being measured randomly for each line. All filled grains from a single plant were collected and dried at 50 °C in an oven for measurement of grain yield per plant. Randomly picked filled grains were used for 1000-grain weight measurements. Total plot grains (randomized block design) were collected in Hangzhou (September 20th, 2018) and Hainan (April 20th, 2019), with two replicates, and treated as described above for measurement of actual yield. Paddy field experiments were fertilized with urea (180 kg N ha −1 ), applied at 60% as basal fertilizer and 40% once during top-dressing per growing season. Reporting summary Further information on research design is available in the Nature Research Reporting Summary linked to this article.